Strongly underestimated dispersion energy in cryptophanes and their complexes Cryptophanes, composed of two bowl-shaped cyclotriveratrylene subunits linked by three aliphatic linker groups, are prototypal organic host molecules which bind reversibly neutral small guest compounds via London forces. The binding constants for these complexes are usually measured in tetrachloroethane and are in the range of 10 2 –10 3 M −1 . Here we show that tetrachloroethane is—in contrast to the scientific consensus—enclosed by the cryptophane-E cavity. By means of NMR spectroscopy we show that the binding constant for CHCl 3 @cryptophane-E is in larger solvents two orders of magnitudes higher than the one measured before. Ab initio calculations reveal that attractive dispersion energy is responsible for high binding constants and for the formation of imploded cryptophanes which seem to be more stable than cryptophanes with empty cavities. Molecular recognition is required for numerous processes in chemistry and biology. Of high interest are noncovalent host-guest interactions which are mainly dominated by London forces [1] , [2] , [3] , [4] , [5] , [6] . The latter are considered as weak molecular interactions and increase with the size of the interacting moieties. The design of host molecules which efficiently bind small nonpolar guests is a great challenge as dispersion interactions of small guests are less intense owing to their small number of atoms. For binding such guests cage compounds are most suitable as they are able to fully enclose molecules and thereby increase the quantity of dispersion interactions [7] , [8] , [9] . Prominent examples for cage compounds are cryptophanes [10] , [11] , [12] . Cryptophanes are composed of two bowl-shaped cyclotriveratrylene (CTV) subunits connected by three aliphatic linker groups, thus forming an interior cavity. Numerous studies have been published which deal with the reversible binding of cryptophane hosts to small nonpolar molecules [12] . Interaction intensities and thus binding constants are highly dependent on the size and shape of the guests and host cavities. By NMR studies it was shown that D 3 -symmetric cryptophane-A ( D 3 - 2 , see Fig. 1 ) forms stable complexes with methane, chloroform and xenon [13] , [14] . Association constants were determined in 1,1,2,2-tetrachloroethane and amount to 130 M −1 for methane and to 230 M −1 for chloroform at 298 K (ref. 13 ). For xenon an even higher binding constant of 3,000 M −1 is found [14] . Here 1,1,2,2-tetrachloroethane was again used as the solvent. It was assumed to be too big to fit into the host cavity, ensuring that the solvent cannot exchange with guest, and that, consequently, the host cavity is empty if no guest is added. If water is used as solvent, the binding constants can be drastically increased. For example, a water-soluble triacetate-functionalized cryptophane-A derivative shows the highest affinity for xenon which was ever measured for a host molecule ( K i =33,000 M −1 at 293 K in buffer) [15] . This increase is explained by entropic (hydrophobic) effects that likely involve desolvation of xenon clathrates upon complexation. An increase of the binding constant can also be observed when the cavity is adjusted to the guest [16] . The D 3 -symmetric cryptophane-E ( D 3 - 1 , see Fig. 1 ) has a slightly larger cavity than cryptophane-A and therefore binds chloroform with a higher association constant ( K i =470 M −1 at 300 K in C 2 D 2 Cl 4 ) [17] , [18] . 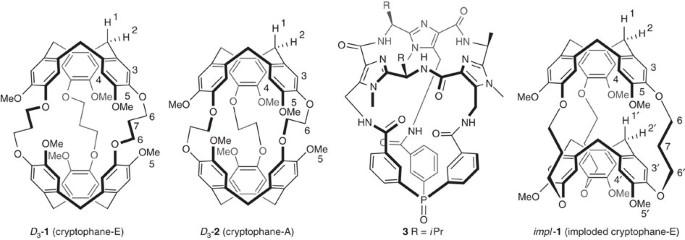Figure 1: Host molecules. Structures of cryptophane-E (D3-1), cryptophane-A (D3-2), the imidazole-containing container3and imploded cryptophane-E (impl-1). Figure 1: Host molecules. Structures of cryptophane-E ( D 3 - 1 ), cryptophane-A ( D 3 - 2 ), the imidazole-containing container 3 and imploded cryptophane-E ( impl - 1 ). Full size image Recently, we were able to show that modified marine cyclopeptides, which are structurally similar to CTVs, can be synthesized in a few steps [19] , [20] , [21] . Structural investigations of modified marine cyclopeptides revealed that small-halogenated hydrocarbons, such as methylene chloride or chloroform, are enclosed into the solid [22] , [23] , [24] . One of these azole-containing cyclopeptides is the C 3 -symmetric cavitand 3 ( Fig. 1 ) which forms a very strong complex with chloroform and other trihalomethanes [25] . As the equilibrium is so strongly shifted to the side of the complex, the thermodynamic parameters of the complex CHCl 3 @ 3 were determined by temperature-dependent NMR spectroscopy at temperatures between 353 and 398 K in 1,1,2,2-C 2 D 2 Cl 4 . From the enthalpy (Δ H i ) and entropy (Δ S i ) of inclusion determined at these temperatures it was possible to calculate the free enthalpy of inclusion (Δ G i ) and hence the binding constant at 300 K. At this temperature K i amounts to 140,000 M −1 for CHCl 3 @ 3 and is thus two orders of magnitude higher than the binding constants for CHCl 3 @ 1 and CHCl 3 @ 2 , respectively. One explanation for this huge difference is probably the fact that chloroform perfectly fits to the shape of the trigonal bipyramidal cavity of 3 , resulting in a multitude of dispersion interactions between the chloroform molecule and the atoms of the cavity. Furthermore, we speculated that a further possible reason for the high stability of CHCl 3 @ 3 compared with that of CHCl 3 @ 1 and CHCl 3 @ 2 may be that the cryptophanes do not completely exclude the solvent, while the container 3 shows improved size discrimination [25] . Here we describe the reinvestigation of cryptophane–guest complexes and focus on the question to which extent C 2 H 2 Cl 4 is enclosed by the cavity. As a representative example we chose the CHCl 3 @cryptophane-E complex (CHCl 3 @ 1 ). By quantum chemical calculations and NMR spectroscopy we show that the solvent is also bound within the cavity and that the binding constant for CHCl 3 @ 1 is two orders of magnitude higher than measured before. Cryptophanes with empty cavities are just reactive intermediates which turn over to more stable forms, the so-called imploded cryptophanes. Determination of the binding constants The assumption that—in contrast to the scientific consensus—C 2 H 2 Cl 4 is also enclosed by cryptophanes can be proven by binding constant determination of cryptophane-E ( D 3 - 1 ) with chloroform in different solvents. If the solvents are enclosed as well, lower binding constants of chloroform should be obtained in these solvents. Crystals containing cryptophane-E and chloroform in a ratio of 1:2 were measured in different deuterated solvents (C 2 D 2 Cl 4 , C 6 D 5 Cl, C 6 D 5 Br and 1,2-C 6 D 4 Cl 2 ) at varying concentrations ( Fig. 2 , Table 1 and Supplementary Figs 1–3 ). In decalin, which is even larger, CHCl 3 @cryptophane-E was not soluble. 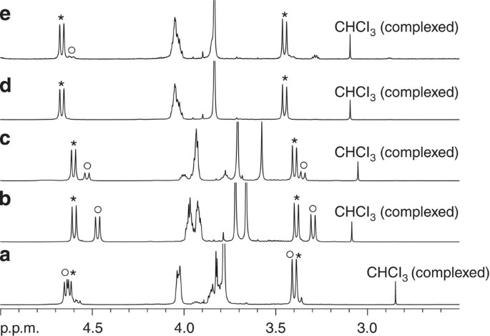Figure 2: Cryptophane-E and CHCl3@cryptophane-E in different solvents. Part of the1H NMR spectra of cryptophane-E (1) without included chloroform and CHCl3@cryptophane-E at 600 MHz in C2D2Cl4(a), C6D5Cl (b), C6D5Br (c), and C6D4Cl2(dande) at 298 K. The sum of the concentrations of1without included chloroform and CHCl3@1amounts to 1.79 mM−1(a), 1.46 mM−1(b), 2.46 mM−1(c), 0.835 mM−1(d) and 0.104 mM−1(e). Stars denote protons H1 and H2 of CHCl3@1, and circles stand for the signals of protons H1 and H2 of1without included chloroform (for numbering seeFig. 1). Figure 2: Cryptophane-E and CHCl 3 @cryptophane-E in different solvents. Part of the 1 H NMR spectra of cryptophane-E ( 1 ) without included chloroform and CHCl 3 @cryptophane-E at 600 MHz in C 2 D 2 Cl 4 ( a ), C 6 D 5 Cl ( b ), C 6 D 5 Br ( c ), and C 6 D 4 Cl 2 ( d and e ) at 298 K. The sum of the concentrations of 1 without included chloroform and CHCl 3 @ 1 amounts to 1.79 mM −1 ( a ), 1.46 mM −1 ( b ), 2.46 mM −1 ( c ), 0.835 mM −1 ( d ) and 0.104 mM −1 ( e ). Stars denote protons H1 and H2 of CHCl 3 @ 1 , and circles stand for the signals of protons H1 and H2 of 1 without included chloroform (for numbering see Fig. 1 ). Full size image Table 1 Thermodynamic data determined by 1 H NMR spectroscopy. Full size table The inclusion of chloroform is strongly dependent on the solvent; in C 2 D 2 Cl 4 , C 6 D 5 Cl and C 6 D 5 Br a CHCl 3 @cryptophane-E/cryptophane-E ratio from 1:1 to 8:1 is found at millimolar host and guest concentrations. The corresponding binding constants amount from 250 to 940 M −1 . As already reported [26] the value in C 2 D 2 Cl 4 is significantly lower than the one published by Collet and collegues [18] . This can probably be ascribed to the inaccuracy of determining the chloroform-free cryptophane-E concentration. The error presumably amounts to ±20%. In 1,2-dichlorobenzene at millimolar host and guest concentrations the CHCl 3 @cryptophane-E complex exists exclusively. Further dilution to 10 −4 and 10 −5 M −1 leads to NMR signal sets (800 scans) of cryptophane-E without enclosed chloroform ( Fig. 2 ; Supplementary Fig. 3 ). The complex formation constant in 1,2-dichlorobenzene amounts to 26,000 M −1 . The impressive difference in the complex formation constants depending on the solvent used shows that the solvent has to be a part of the equilibrium. One possible interpretation is—as already assumed [25] —that the solvent can also be enclosed by cryptophane-E. Larger solvent molecules like 1,2-C 6 D 4 Cl 2 are less effectively enclosed and therefore lead to higher chloroform binding constants, whereas solvents like C 2 D 2 Cl 4 show lower CHCl 3 @ 1 binding constants. Thus, measurements in such solvents significantly underestimate the binding capability of cryptophanes. Imploded cryptophane-E Following the above argument the NMR signals for cryptophane-E without chloroform should not be derived from empty cryptophane-E, but from solvent@cryptophane-E. We thus had to find out if the empty cryptophane can also be observed by NMR measurements because this would be a proof for the solvent@cryptophane-E complexes. For this purpose the NMR samples were heated stepwise to 378 K, as higher temperatures should favour the exclusion of chloroform and the solvent, so that an empty container is generated owing to entropy gain. However, increased temperatures lead to faster molecule exchange and thus just one set of NMR signals for cryptophane-E and its chloroform complex are observed at temperatures higher than 338 K ( Fig. 3 ; Supplementary Figs 4 and 5 ). But at 338 K and above there is one additional set of signals pointing to a C 3 -symmetric-imploded cryptophane-E ( impl - 1 ; see Fig. 1 ). After cooling to 298 K both signal sets (for cryptophane-E with and without chloroform) reoccur and the additional set of signals for the imploded cryptophane-E is also visible. At 298 K the transformation of impl - 1 to the solvent@ 1 complex takes place very slowly (several days). 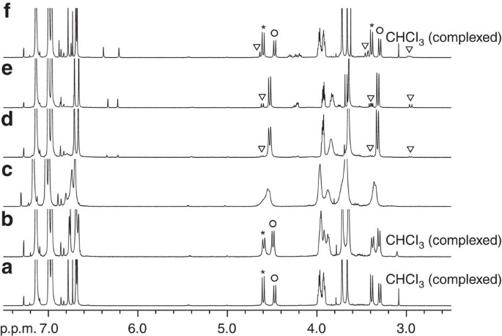Figure 3: Cryptophane-E and CHCl3@cryptophane-E in C6D5Cl at different temperatures. 1H NMR spectra of cryptophane-E (D3-1) without included chloroform and CHCl3@cryptophane-E at 600 MHz in C6D5Cl at 298 K (a), 318 K (b), 338 K (c), 358 K (d), 378 K (e) and after cooling to 298 K (f). Stars denote protons H1 and H2 of CHCl3@1, circles stand for the signals of protons H1 and H2 ofD3-1without included chloroform, and triangles mark protons H1, H1′, H2 and H2′ of the imploded cryptophane-E (impl-1) (for numbering seeFig. 1). Figure 3: Cryptophane-E and CHCl 3 @cryptophane-E in C 6 D 5 Cl at different temperatures. 1 H NMR spectra of cryptophane-E ( D 3 - 1 ) without included chloroform and CHCl 3 @cryptophane-E at 600 MHz in C 6 D 5 Cl at 298 K ( a ), 318 K ( b ), 338 K ( c ), 358 K ( d ), 378 K ( e ) and after cooling to 298 K ( f ). Stars denote protons H1 and H2 of CHCl 3 @ 1 , circles stand for the signals of protons H1 and H2 of D 3 - 1 without included chloroform, and triangles mark protons H1, H1′, H2 and H2′ of the imploded cryptophane-E ( impl - 1 ) (for numbering see Fig. 1 ). Full size image The occurrence of one C 3 -symmetric set of signals for impl - 1 can either mean that impl - 1 adopts a C 3 -symmetric in-out conformation or that it exhibits a C 1 -symmetric out-saddle conformation [12] which leads to a C 3 -symmetric spectrum owing to pseudorotation [27] . The latter conformation has already been described for cryptophane-A derivatives and larger cryptophanes [16] , [28] , [29] . To determine the conformation of impl - 1 , a mixture of CHCl 3 @ 1 in 1,2-C 6 D 4 Cl 2 was heated at 423 K for 12 h to completely remove CHCl 3 from the solution. In a second experiment CHCl 3 @ 1 in C 6 D 5 Cl was heated at 393 K for 12 h. Both experiments resulted in a 2:1 mixture of impl - 1 and solvent@ 1 which was analysed by variable temperature and two-dimensional nuclear Overhauser enhancement spectroscopy (NOESY) experiments. The NOESY spectra show no distinct cross peaks between the protons of opposite CTV units. In the temperature-dependent NMR spectra the signal for proton H1′ becomes broader owing to decreasing temperature ( Supplementary Figs 6 and 7 ). Both results suggest a dynamic process which unambiguously points to the C 1 -symmetric out-saddle conformation of impl - 1 . Proof of the inclusion of C 2 H 2 Cl 4 into cryptophane-E To deliver a direct proof that 1,1,2,2-C 2 H 2 Cl 4 is enclosed by cryptophane-E we decided to analyse a mixture of C 2 H 2 Cl 4 @ 1 and CHCl 3 @ 1 in C 2 H 2 Cl 4 with ca . 9% of C 2 D 2 Cl 4 . The occurrence of a highfield-shifted signal for the protons of C 2 H 2 Cl 4 in C 2 H 2 Cl 4 @ 1 should be a proof for the formation of C 2 H 2 Cl 4 @ 1 . The strong solvent signal of C 2 H 2 Cl 4 in the 1 H NMR spectrum made it necessary to use higher concentrations of CHCl 3 @ 1 . However, this higher concentration leads to the existence of only CHCl 3 @ 1 ( Supplementary Fig. 8 ). To completely remove the chloroform the solution was heated at 413 K for 20 h. In the resulting solution, exclusively the signals for C 2 H 2 Cl 4 @ 1 and impl - 1 are found. The signal for enclosed C 2 H 2 Cl 4 can be found at 1.58 p.p.m. ( Supplementary Fig. 9 ). An unambiguous proof that this signal indeed belongs to the enclosed solvent can be found in the NOESY spectrum, which exhibits a cross peak between free C 2 H 2 Cl 4 at 5.99 p.p.m. and enclosed C 2 H 2 Cl 4 at 1.58 p.p.m. ( Fig. 4 ). To verify that this signal is no artefact caused by the high concentration of nondeuterated solvent, the NOESY spectrum was monitored using a different spectrometer frequency (600 MHz). At this frequency the exchange signal can also be observed. 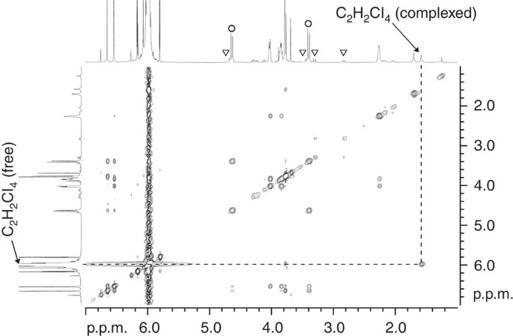Figure 4: NOESY NMR spectrum of C2H2Cl4@1 and imploded cryptophane-E. 1H–1H NOESY NMR spectrum of C2H2Cl4@1andimpl-1at 500 MHz in C2H2Cl4/C2D2Cl4(10:1) at 298 K. The cross peak between the complexed C2H2Cl4and the free C2H2Cl4is highlighted. Circles denote protons H1 and H2 of C2H2Cl4@1, and triangles stand for protons H1, H1′, H2 and H2′ ofimpl-1(for numbering seeFig. 1). Figure 4: NOESY NMR spectrum of C 2 H 2 Cl 4 @1 and imploded cryptophane-E. 1 H– 1 H NOESY NMR spectrum of C 2 H 2 Cl 4 @ 1 and impl - 1 at 500 MHz in C 2 H 2 Cl 4 /C 2 D 2 Cl 4 (10:1) at 298 K. The cross peak between the complexed C 2 H 2 Cl 4 and the free C 2 H 2 Cl 4 is highlighted. Circles denote protons H1 and H2 of C 2 H 2 Cl 4 @ 1 , and triangles stand for protons H1, H1′, H2 and H2′ of impl - 1 (for numbering see Fig. 1 ). Full size image Further investigations were made to prove the exchange signal utilising rotating-frame Overhauser effect spectroscopy (ROESY) and selective ROESY techniques, which are ideally suited for identifying chemical exchange processes [30] . The sign of the cross peak immediately discriminates between cross relaxation chemical exchange types of magnetisation transfer. As expected a negative sign is found for the cross signal of the protons at 5.99 and 1.58 p.p.m., whereas NOE cross peaks (for example, the cross peaks of protons H1 and H2; see Supplementary Figs 10 and 11 ) exhibit positive signs. Further evidence for the inclusion of C 2 H 2 Cl 4 is delivered by the 1 H– 13 C correlation spectroscopy NMR spectrum, in which a cross peak between the hydrogen of the complexed C 2 H 2 Cl 4 and the carbon of the complexed C 2 H 2 Cl 4 appears ( Supplementary Fig. 12 ). Calculation of the cryptophanes and their complexes To evaluate the contribution of attractive dispersion forces to the energy of the inclusion, ab initio calculations were carried out. The molecular structures of the cryptophanes and their complexes were optimized using the density functional theory (DFT) potential M05-2X which has been shown to cover midrange correlation [31] . For the light elements C, H and O the 6-31G* basis set was used, whereas for the halogens Cl and Br the cc-pVTZ basis set was employed. The calculation results are summarized together with the ones obtained for the imidazole-containing container 3 in Table 2 ( Fig. 5 , Supplementary Fig. 13 , Supplementary Table 1 and Supplementary Data 1 ). A comparison of the calculated (M05-2X) interaction energies of different cryptophane-E complexes shows that in accordance with the experiments the inclusion of all chosen solvent molecules is possible. The difference of gas phase complex formation energies between CHCl 3 @ 1 and C 2 H 2 Cl 4 @ 1 is just marginal (1.4 kcal mol −1 ). The experimentally determined preference of CHCl 3 @ 1 complex formation in C 2 H 2 Cl 4 has thus to be ascribed for entropic reasons. Even for the smaller cryptophane-A the inclusion of C 2 H 2 Cl 4 is energetically possible. Only for imidazole-containing container 3 the inclusion of C 2 H 2 Cl 4 leads to an energetic destabilization of the system. Table 2 Calculated interaction energies. 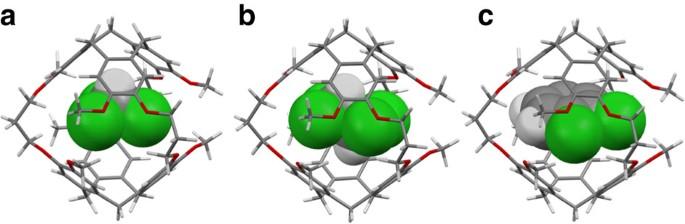Figure 5: Molecular structures of inclusion complexes of cryptophane-E. The geometry of the complexes CHCl3@1(a), C2H2Cl4@1(b) and C6H4Cl2@1(c) was optimized using M05-2X/6-31G*,cc-pVTZ. Full size table Figure 5: Molecular structures of inclusion complexes of cryptophane-E. The geometry of the complexes CHCl 3 @ 1 ( a ), C 2 H 2 Cl 4 @ 1 ( b ) and C 6 H 4 Cl 2 @ 1 ( c ) was optimized using M05-2X/6-31G*,cc-pVTZ. Full size image Figure 5 depicts the calculated (M05-2X) structures of cryptophane-E ( D 3 - 1 ) with different guests. It is evident that despite different guests the cryptophane-E host structures of all complexes do not vary significantly. The distances between the middle CH 2 -propane groups in the complexes amount to 10.33 Å on average (10.27 Å for CHCl 3 @ 1 , 10.35 Å for C 2 H 2 Cl 4 @ 1 and 10.38 Å for C 6 H 4 Cl 2 @ 1 ) and the distances between the methylene groups of opposite CTV units are 9.91 Å on average (9.91 Å for CHCl 3 @ 1 , 9.92 Å for C 2 H 2 Cl 4 @ 1 and 9.91 Å for C 6 H 4 Cl 2 @ 1 ). The guests are oriented in such a way that the large atoms (chlorine) preferably lie within the plane formed by the middle CH 2 -propane groups. Based on the geometries obtained by M05-2X/6-31G*,cc-pVTZ, single point calculations with B3LYP [32] , [33] , [34] and B3LYP-D3 were carried out. While the first method cannot describe the dispersion interaction correctly, especially not at large distances, the latter one includes an additional dispersion correction [35] , [36] . Thus, the difference between the two is a hint to the extent of the complex dispersion energies. For the light elements C, H and O the 6-311++G** basis set was used, whereas for the halogens Cl and Br the aug-cc-pVTZ basis set was employed. The data thus obtained are summarized in Table 2 . A comparison of the methods B3LYP and B3LYP-D3 shows that in all cases dispersion interactions are predicted to be the driving force for inclusion. For structural investigations of the imploded cryptophanes a C 1 -symmetric out-saddle conformation of imploded cryptophane-A ( impl - 2 ) [16] , a C 3 -symmetric in-out conformation of imploded cryptophane-E ( impl - 1 ) and a C 1 -symmetric out-saddle conformation of impl - 1 were optimized using M05-2X/6-31G*,cc-pVTZ (see Fig. 6 ). Based on these geometries single point calculations with B3LYP and B3LYP-D3 were carried out ( Table 3 ). The calculations show that the C 1 -symmetric out-saddle conformation of impl - 1 is energetically more favourable than the C 3 -symmetric in-out conformation ( Table 3 ). Without taking the dispersion correction into account (by using the simple B3LYP method) the D 3 -symmetric out-out conformers are much more stable than the corresponding imploded structures. This means that the intramolecular dispersion interactions between the CTV units is predicted to stabilize the imploded structures in contrast to the out-out cavity systems. 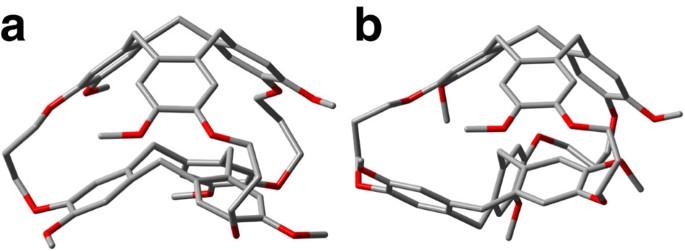Figure 6: Structure of imploded cryptophane-E. Molecular structures of imploded cryptophane-E (impl-1) ((a)in-outconformation; (b)saddle-outconformation) calculated using M05-2X/6-31G*,cc-pVTZ. All hydrogen atoms are omitted for clarity. Figure 6: Structure of imploded cryptophane-E. Molecular structures of imploded cryptophane-E ( impl - 1 ) (( a ) in-out conformation; ( b ) saddle-out conformation) calculated using M05-2X/6-31G*,cc-pVTZ. All hydrogen atoms are omitted for clarity. Full size image Table 3 Calculated relative gas phase energies. Full size table We have shown that—in contrast to the scientific consensus—cryptophanes are able to enclose bigger solvent molecules. Because of this inclusion the complex formation constants for cryptophane–guest complexes measured previously have been underestimated. If a solvent like 1,2-dichlorobenzene is used, which is enclosed less effectively by the cryptophane-E cavity, the binding constant for CHCl 3 @cryptophane-E is two orders of magnitude higher. The reason for these high binding constants is predicted by the DFT simulations to be strong dispersion interactions. Using the B3LYP method an energetic stabilisation cannot be found for any guest. Only if the dispersion correction D3 is added, energetic stabilisation can be found. These corrections reach values from 25 to 46 kcal mol −1 . As the dispersion interactions increase with the number of interacting atoms, a comparison is only reasonable if the dispersion correction for each interacting atom is regarded. The highest values are found for the chloroform complexes (7.8 kcal for CHCl 3 @ 1 , 8.3 kcal for CHCl 3 @ 2 and 8.5 kcal for CHCl 3 @ 3 ). It has to be considered though that only the interaction energy during the inclusion of the halogen compounds into the cavity is calculated. It is not possible to make any statement with respect to solvent interaction and entropic factors. The inclusion of larger molecules like 1,1,2,2-tetrachloroethane and 1,2-dichlorobenzene, which according to experiments are disfavoured compared with chloroform binding, presumably leads to a high loss of entropy as the motion of the enclosed molecules is restricted. The calculations also explain the fact that CHCl 3 @ 3 in C 2 H 2 Cl 4 exhibits a complex formation constant which is two magnitudes higher than that of CHCl 3 @ 1 in C 2 H 2 Cl 4 : while the inclusion of solvent can be excluded by energetic reasons for compound 3 , cryptophane-E is able to enclose solvent molecules. The occurrence of a C 1 -symmetric out-saddle conformation of impl - 1 at higher temperatures implies that the empty host compound D 3 - 1 is quite unstable: The empty cryptophane-E either turns into the stable impl - 1 form or immediately encloses a guest leading to the complex solvent@cryptophane-E. DFT calculations predict that intramolecular dispersion interactions between the CTV units are responsible for the fact that cryptophanes with empty cavities are only reactive intermediates. If no guest is enclosed, the more stable form is the corresponding imploded cryptophane. Computational study All calculations were performed by using the programme package Gaussian 09 (ref. 37) [37] and MOLPRO [38] . Geometry optimizations were performed using the DFT potential M05-2X [31] . For the light elements C, H and O the 6-31G* basis set was used, whereas for the halogens Cl and Br the cc-pVTZ basis set was employed. Compounds 1 and CHCl 3 @ 1 were completely geometrically optimized within the C 3 point group. All other compounds were optimized without any symmetry restriction. For the cryptophane-A and its complexes the gauche, trans, trans conformation of the -O-CH 2 -CH 2 -O-bridges was taken, because this one is also found in the solid state [39] . To determine the structure of impl - 1 several C 3 -symmetric in-out conformations of imploded cryptophane-E ( impl - 1 ) and several C 1 -symmetric out-saddle conformations of impl - 1 were optimized using M05-2X/6-31G*,cc-pVTZ. The conformers only vary in the conformation of the three propane bridges. Only the most stable in-out and out-saddle conformer are given in Table 3 . Based on the geometries obtained by M05-2X/6-31G*,cc-pVTZ, single point calculations with B3LYP [32] , [33] , [34] and B3LYP-D3 (refs 35 , 36 ) were carried out. For the light elements C, H and O the 6-311++G** basis set was used, whereas for the halogens Cl and Br the aug-cc-pVTZ basis set was employed. See Supplementary Table 1 and Supplementary Data 1 . Experimental section Cryptophane-E was synthesized according to literature procedures [40] . To guarantee that no undesired small solvent molecules are enclosed by the cryptophane, a big charge of cryptophane-E was firstly recrystallized from acetone and secondly from chloroform. Subsequent NMR measurements showed that the obtained crystals feature a cryptophane-E/chloroform ratio of 1:2. This ratio was also found by X-ray structure analysis of the solid [18] . 1 H, 13 C NMR and 2D NMR spectra were measured with Bruker Avance DRX 500 and HD 600 spectrometers. Characterisation data of cryptophane-E ( 1 ): mp. 308.5 °C; 1 H NMR (600 MHz, CDCl 3 ): δ=6.69 (s, 6H, H ar ), 6.61 (s, 6H, H ar ), 4.66 (d, 2 J H,H =13.7 Hz, 6H, CH 2 ), 4.06 (m, 6H, CH 2 ), 3.88 (m, 6H, CH 2 ), 3.83 (s, 18H, OCH 3 ), 3.43 (d, 2 J H,H =13.8 Hz, 6H, CH 2 ), 2.31 (m, 6H, CH 2 ) p.p.m. ; 13 C NMR (151 MHz, CDCl 3 ): δ=147.10 (q, C ar ), 131.01 (q, C ar ), 130.96 (q, C ar ), 112.27 (t, C ar ), 112.03 (t, C ar ), 63.60 (s, CH 2 ), 55.62 (p, OCH 3 ), 36.10 (s, CH 2 ), 29.65 (s, CH 2 ) p.p.m. ; IR (ATR): =2,990, 2,861, 1,608, 1,511, 1,470, 1,444, 1,399, 1,343, 1,257, 1,215, 1,193, 1,139, 1,084, 1,054, 1,020, 981, 941, 873, 851, 750, 667 cm −1 ; UV/Vis (dichloromethane): λ max (log ε )=290 (3.66), 232 (4.11), 208 (4.40) nm; high-resolution mass spectrometry (electrospray ionization-positive) ( m/z ): [M+Na] + calculated for C 57 H 60 NaO 12 , 959.3983; found, 959.3971. How to cite this article: Haberhauer, G. et al. Strongly underestimated dispersion energy in cryptophanes and their complexes. Nat. Commun. 5:3542 doi: 10.1038/ncomms4542 (2014).